Generation and characterization of influenza A viruses with altered polymerase fidelity Genetic diversity of influenza A viruses (IAV) acquired through the error-prone RNA-dependent RNA polymerase (RdRP) or through genetic reassortment enables perpetuation of IAV in humans through epidemics or pandemics. Here, to assess the biological significance of genetic diversity acquired through RdRP, we characterize an IAV fidelity variant derived from passaging a seasonal H3N2 virus in the presence of ribavirin, a purine analogue that increases guanosine-to-adenosine mutations. We demonstrate that a single PB1-V43I mutation increases selectivity to guanosine in A/Wuhan/359/95 (H3N2) and A/Vietnam/1203/04 (H5N1) viruses. The H5N1 PB1-V43I-recombinant virus replicates to comparable titres as the wild-type virus in vitro or in the mouse lungs. However, a decrease in viral population diversity at day 3 post inoculation is associated with a tenfold reduced lethality and neurotropism in mice. Applying a fidelity variant with reduced mutational frequency, we provide direct experimental evidence for the role of genetic diversity in IAV pathogenesis. The mechanisms for generating influenza A virus (IAV) genetic diversity are its RNA-dependent RNA polymerase (RdRP) that lacks a proof-reading mechanism and its segmented genome that facilitate genetic reassortment between different IAVs. Thus, as with other RNA viruses, influenza viruses exist as a population of genetic variants, and such diversity cannot be assessed by the consensus sequence [1] , [2] . Such a genetic diversity allows adaptation of an RNA virus to different selection pressure as exemplified by the antigenic drift variants that emerge from a plethora of genetic variants when selected under immune pressure [2] , [3] , [4] . However, the molecular mechanisms by which the IAV polymerase contributes to viral genetic diversity and how such diversity affects pathogenicity in vivo remain poorly studied [2] . Ribavirin (1-[(2R,3R,4S,5R)-3,4-dihydroxy-5-(hydroxymethyl)oxolan-2-yl]-1H-1,2,4-triazole-3-carboxamide), a purine analogue, inhibits replication of RNA viruses by different mechanisms, including the depletion of the cellular GTP pool by competing with cellular inosine monophosphate for inosine monophosphate dehydrogenase, interfering with RNA capping, inhibiting RdRP or by acting as a mutagen leading to lethal mutagenesis [5] , [6] , [7] . As a mutagen, ribavirin has been used to select high-fidelity variants of positive-sense, single-stranded RNA viruses of the Piconaviridae and Togaviridae families [8] , [9] , [10] , [11] with similar RdRP structures [12] . In contrast, IAV possesses a heterotrimeric polymerase complex formed by the PB2, PB1 and PA proteins with the RdRP catalytic function residing in the PB1 protein [13] . The molecular workings of its polymerase, including fidelity, are poorly understood, and it is not known if ribavirin can induce mutagenesis in the IAV genome. Favipiravir (T-705), a novel antiviral drug and a purine analogue with a broad antiviral polymerase activity, has recently been shown to induce mutagenesis in the influenza genome [14] . Here, to gain insights into the biological significance of IAV mutation frequency and viral genetic diversity on viral pathogenesis, we generate influenza RdRP fidelity variants by the serial passage of a human seasonal H3N2 influenza virus (A/Wuhan/359/95; Wuhan95) in the presence of ribavirin. We confirm that ribavirin functions as a mutagen for IAV by increasing G-to-A and C-to-T mutations in vitro . PB1-V43I mutation is identified to increase polymerase fidelity in recombinant Wuhan95 virus as well as in a highly pathogenic H5N1 virus (A/Vietnam/1203/04; VN04). The recombinant VN04 virus with the PB1-V43I mutation replicates to comparable titres as the wild-type counterpart in vitro or in the mouse lungs, but has reduced population diversity at day 3 post inoculation. Such reduced genetic diversity at an early time point post infection is associated with a reduced lethality and neurovirulence. Our results identify a single V43I mutation in PB1 protein that affects viral genetic diversity and provide the first experimental evidence of the role of genetic diversity in IAV pathogenicity. Mutagenic effects of ribavirin on IAV genome We first determined whether ribavirin can induce mutagenesis in the IAV genome. To determine the effect of ribavirin on IAV genomic mutational frequencies, recombinant virus Wuhan95 (H3N2) was passaged four times in the presence (35 μM) or absence of ribavirin and the HA1 gene was analysed by clonal sequencing. 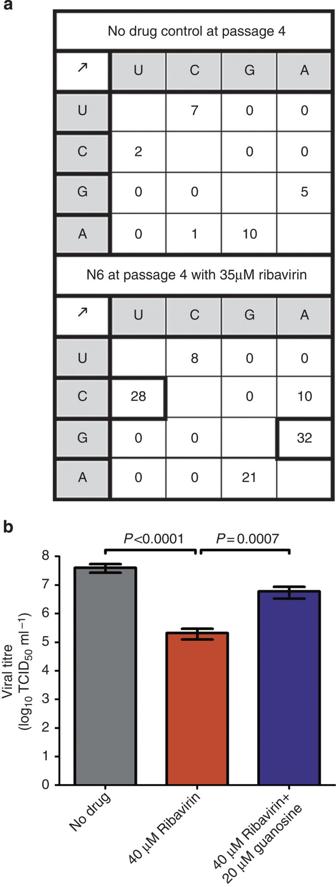Figure 1: The mutagenic effect of ribavirin on IAV genome. (a) Frequencies of nucleotide substitutions in theHA1gene (nts 140–883, numbering from ATG) of Wuhan95 viruses that were serial passaged four times in the absence (no drug control) or presence (N6) of 35 μM ribavirin in MDCK cells. Six clones for N6 and two clones for no drug control were analysed. Nucleotide changes from letters in the first column to those in the first row were shown, with the most frequent changes highlighted in the black boxes. Increased G-to-A and C-to-T mutations were noted in N6 after four passages in the presence of ribavirin (Fisher’s exact test,P=0.0010). Fisher’s exact test was based on a 2 × 2 contingency table constructed to compare the relative number of G-to-A mutations to A-to-G mutations between wild-type and V43I viruses. (b) Ribavirin competition assay with nucleoside guanosine was performed with the Wuhan95 virus at MOI=0.1 in MDCK cells under three different conditions: no drug treatment, 40 μM of ribavirin and 40 μM ribavirin plus 20 μM guanosine. Culture supernatants were harvested at 48 h post infection to determine viral titres (log10TCID50per ml). Student’st-test was performed to compare the difference in viral titres between different treatment groups. The mean viral titers±s.d. from triplicates derived from one out of two independent experiments are shown. After four serial passages in vitro , ribavirin increased genomic mutation frequency from 3.69 (25 out of 67,704) to 15.74 (89 out of 56,544) per 10 4 nucleotide sequenced (Fisher’s exact test, P <0.0001; Supplementary Table 1 ), predominantly with the characteristic G-to-A and complementary C-to-T mutations (Fisher’s exact test, P =0.001; Fig. 1a ). This observation suggested that the purine analogue ribavirin can cause mutagenesis in the IAV genome. We then evaluated whether addition of guanosine may compete with ribavirin and rescue viral replication. First, the 50% cytotoxic concentration (CC 50 ) of guanosine and ribavirin in Madin-Darby canine kidney (MDCK) cells was determined by MTT (3-(4,5-dimethylthiazol-2-yl)-2,5-diphenyltetrazolium bromide) assay to be 122.00±0.11 μM (mean CC 50 ±s.e. ; Supplementary Fig. 1a ) and 352.00±0.04 μM, respectively ( Supplementary Fig. 1b ). In the presence of 40 μM ribavirin, we observed that the addition of 20 μM guanosine reversed the inhibition of Wuhan95 by ribavirin ( Fig. 1b ). This confirms previous observations that guanosine can reverse the antiviral activity of ribavirin at non-cytotoxic concentrations for influenza virus [15] , [16] , [17] , [18] . Thus, although ribavirin can inhibit RdRP directly [16] , our data shows that ribavirin can also cause mutagenesis in the IAV genome as a purine analogue. Figure 1: The mutagenic effect of ribavirin on IAV genome. ( a ) Frequencies of nucleotide substitutions in the HA1 gene (nts 140–883, numbering from ATG) of Wuhan95 viruses that were serial passaged four times in the absence (no drug control) or presence (N6) of 35 μM ribavirin in MDCK cells. Six clones for N6 and two clones for no drug control were analysed. Nucleotide changes from letters in the first column to those in the first row were shown, with the most frequent changes highlighted in the black boxes. Increased G-to-A and C-to-T mutations were noted in N6 after four passages in the presence of ribavirin (Fisher’s exact test, P =0.0010). Fisher’s exact test was based on a 2 × 2 contingency table constructed to compare the relative number of G-to-A mutations to A-to-G mutations between wild-type and V43I viruses. ( b ) Ribavirin competition assay with nucleoside guanosine was performed with the Wuhan95 virus at MOI=0.1 in MDCK cells under three different conditions: no drug treatment, 40 μM of ribavirin and 40 μM ribavirin plus 20 μM guanosine. Culture supernatants were harvested at 48 h post infection to determine viral titres (log 10 TCID 50 per ml). Student’s t -test was performed to compare the difference in viral titres between different treatment groups. The mean viral titers±s.d. from triplicates derived from one out of two independent experiments are shown. Full size image Isolating H3N2 variants with reduced ribavirin sensitivity Since ribavirin was observed to increase IAV RdRP mutational frequency, we hypothesized that the selection of an IAV ribavirin-resistant variant may yield an RdRP fidelity variant as reported previously for other RNA viruses [9] , [19] , [20] . We serially passaged a human seasonal H3N2 influenza strain Wuhan95 (H3N2) in six replicates in MDCK cells at a constant multiplicity of infection (MOI) of 0.01 TCID 50 per cell from passages 1 to 11 in the presence of 35 μM ribavirin. This concentration of ribavirin was previously determined to be at approximately EC 75 by determining viral titre from culture supernatant ( Supplementary Fig. 2a ) and by determining M gene copy numbers using quantitative real-time PCR ( Supplementary Fig. 2b ). After 11 serial passages in the presence of 35 μM ribavirin, we raised the concentration of ribavirin to 40μM and continued passaging the virus for six more passages, aiming to isolate variants that can replicate at a higher concentration of ribavirin and to further increase the proportion of ribavirin-resistant variant in the total virus population. Two of the six replicates, N1 and N6, went extinct at passage 5 as no virus progeny can be detected using TCID 50 assay (detection limit=1.789 log 10 TCID 50 per ml; Supplementary Fig. 2c ). Two more replicates, N3 and N5, subsequently went extinct at passage 12. Replicates N2 and N4 were passaged in the presence of ribavirin until passage 17 ( Supplementary Fig. 2c ), at which point plaque reduction assays were performed to isolate virus clones with increased resistance to ribavirin. A total of 182 plaques that showed reduced sensitivity at 40 μM ribavirin in plaque reduction assay were picked and were expanded once in the absence of ribavirin before further testing for their sensitivity to ribavirin by plaque reduction assay. Six expanded clones derived from replicate N4 and two clones from replicate N2 that showed a consistently reduced sensitivity to ribavirin were selected for Sanger sequencing to map potential mutations in PB2 , PB1 , PA and NP genes that may confer to ribavirin resistance. 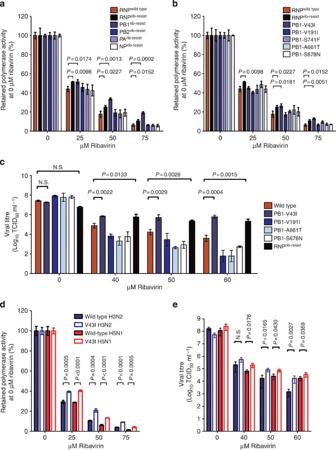Figure 2: Applying polymerase-based mini-genome assay to identify mutation(s) conferring reduced sensitivity to ribavirin. (a) Effect of the gene segment conferring to ribavirin resistance was evaluated by substituting wild-type Wuhan95 polymerase (RNPwild type), withPB1,PB2,PAorNPgenes from the ribavirin-resistant variant (N4) harbouring all 10 mutations (RNPrib-resist). The experiment was performed two times with similar trends. (b) Mapping of the PB1 mutation conferring to ribavirin resistance was performed by substituting each of the five PB1 mutations identified from the ribavirin-resistant clones N4 and N2. The ratio of firefly luciferase and renilla luciferase derived for each reaction was normalized to that of the ratio derived at 0 μM ribavirin (retained polymerase activity %). Three independent experiments were performed with one representative result shown. The error bars represent the s.d. of triplicates (N=3). (c) Ribavirin dose–response curve in MDCK cells using recombinant Wuhan95 viruses each carrying a single-point mutation (V43I, V191I, A661T and S678N) in PB1. Cells were infected at MOI=0.1 and the supernatants were harvested at 48 h post infection for titration. The error bars represent the s.d. determined for triplicates (N=3) for one representative experiment. The experiment was performed two times. One representative result of two independent experiments is shown. (d) Mini-genome assays for polymerase activity were performed in the presence of increasing concentrations of ribavirin to compare the sensitivities of the wild type with the PB1-V43I counterparts using H3N2 or H5N1 polymerase complexes. The error bars represent samples prepared in triplicates (N=3). The experiment was performed three times. (e) Ribavirin dose–response curve in MDCK cells using the recombinant H3N2 and H5N1 viruses with or without the PB1-V43I mutation.Pvalues are based on Student’st-test. N.S. denotes not statistically significant. The error bar represents the s.d. determined from samples prepared in triplicates (N=3). The ribavirin dose–response curve with Wuhan95 (H3N2) wild-type and PB1-V43I-mutant viruses were repeated five times. PB1-V43I confers ribavirin resistance to H3N2 and H5N1 IAV Eleven mutations were identified in genes from the six expanded clones from N4 and two expanded clones from N2 with reduced sensitivity to ribavirin, five mutations in PB1, two in PB2, one in PA and three in NP ( Supplementary Table 2 ). We introduced 10 mutations found in the clones derived from the N4 replicate ( Supplementary Table 2 ) into the PB2 (PB2-D309N, PB2-R702K), PB1 (PB1-V43I, PB1-V191I, PB1-A661T, PB1-S741F), PA (PA-L54F) and NP (NP-D101N, NP-S287N, NP-M371I) proteins as RNP rib-resist ( Fig. 2a ). The PB1-S678N mutation found in the N2 replicate was tested separately ( Fig. 2b ). We used a reductionist approach based on a mini-genome assay to assess the role of each mutation on ribavirin sensitivity. First, we identified that the mutations conferring the ribavirin resistance phenotype resided in PB1, as co-transfecting the PB1 plasmid harbouring the four mutations (V43I, V191I, A661T, S741F) identified from the clones derived from the N4 replicate with the PB2, PA or NP plasmids derived from the wild-type virus exhibited reduced sensitivity to ribavirin ( Fig. 2a ). In reverse, replacing each of the PB2, PB1, PA or NP plasmids derived from RNP rib-resist with that from the wild-type RNP confirm that only retaining the PB1 derived from RNP rib-resist show reduced sensitivity to ribavirin in the mini-genome assay ( Supplementary Fig. 3a ). We then individually evaluated the effect of all the mutations identified in the PB1 of the N2 (S678N) and N4 (V43I, V191I, A661T, S741F) replicates by the mini-genome assay ( Fig. 2b ). S741F mutation was found to confer minimal resistance to ribavirin ( Fig. 2b ) and significantly reduced polymerase activity of Wuhan95 polymerase complex by 2.4-fold ( Table 1 ). Through testing each of the PB1 mutations with the mini-genome assay, we identified the PB1-V43I mutation that exhibited most significant resistance to ribavirin ( Fig. 2b ), with an EC 50 (effector concentration for half-maximum response) value of 95.59 μM (95% confidence interval (CI), 70.92–128.8 μM) while the EC 50 of the wild-type polymerase was 41.67 μM (95% CI, 36.24–47.91 μM; Table 1 ). The PB1-V43I mutation was observed to reduce the polymerase activity of the Wuhan95 virus by 50% by the polymerase-based mini-genome assay ( Table 1 ). Figure 2: Applying polymerase-based mini-genome assay to identify mutation(s) conferring reduced sensitivity to ribavirin. ( a ) Effect of the gene segment conferring to ribavirin resistance was evaluated by substituting wild-type Wuhan95 polymerase (RNP wild type ), with PB1 , PB2 , PA or NP genes from the ribavirin-resistant variant (N4) harbouring all 10 mutations (RNP rib-resist ). The experiment was performed two times with similar trends. ( b ) Mapping of the PB1 mutation conferring to ribavirin resistance was performed by substituting each of the five PB1 mutations identified from the ribavirin-resistant clones N4 and N2. The ratio of firefly luciferase and renilla luciferase derived for each reaction was normalized to that of the ratio derived at 0 μM ribavirin (retained polymerase activity %). Three independent experiments were performed with one representative result shown. The error bars represent the s.d. of triplicates ( N =3). ( c ) Ribavirin dose–response curve in MDCK cells using recombinant Wuhan95 viruses each carrying a single-point mutation (V43I, V191I, A661T and S678N) in PB1. Cells were infected at MOI=0.1 and the supernatants were harvested at 48 h post infection for titration. The error bars represent the s.d. determined for triplicates ( N =3) for one representative experiment. The experiment was performed two times. One representative result of two independent experiments is shown. ( d ) Mini-genome assays for polymerase activity were performed in the presence of increasing concentrations of ribavirin to compare the sensitivities of the wild type with the PB1-V43I counterparts using H3N2 or H5N1 polymerase complexes. The error bars represent samples prepared in triplicates ( N =3). The experiment was performed three times. ( e ) Ribavirin dose–response curve in MDCK cells using the recombinant H3N2 and H5N1 viruses with or without the PB1-V43I mutation. P values are based on Student’s t -test. N.S. denotes not statistically significant. The error bar represents the s.d. determined from samples prepared in triplicates ( N =3). The ribavirin dose–response curve with Wuhan95 (H3N2) wild-type and PB1-V43I-mutant viruses were repeated five times. Full size image Table 1 The effect of the identified PB1 mutations on ribavirin sensitivity and polymerase activity using mini-genome assays. Full size table To confirm the results derived from the mini-genome assay, we generated recombinant H3N2 viruses harbouring each of the four mutations in PB1 (S678N from replicate N2 and V43I, V191I and A661T from replicate N4). The S741F mutation was excluded because it conferred minimal resistance to ribavirin and reduced polymerase activity by mini-genome assay ( Table 1 ). Under increasing concentration of ribavirin, the recombinant Wuhan95 virus carrying the PB1-V43I mutation showed the most pronounced ribavirin resistance with a 10.8-fold higher virus titre at 60 μM ribavirin compared with that of the wild-type-recombinant Wuhan95 virus ( Fig. 2c,e ). The EC 50 value of Wuhan95-recombinant PB1-V43I virus at an MOI of 0.1 was 73.49 μM (95% CI, 60.67–89.03 μM), which is higher than that of the recombinant wild-type virus, with an EC 50 value of 39.49 μM (95% CI, 35.65–43.74 μM). PB1-V43 lies within the putative viral RNA-binding domain in the amino terminus of PB1 and is highly conserved among IAV [21] . To evaluate whether the PB1-V43I mutation would confer resistance to ribavirin in a different IAV polymerase complex, we introduced the V43I mutation into the H5N1 highly pathogenic VN04 virus. We observed that the V43I mutation similarly confers resistance to ribavirin in a mini-genome assay, with an EC 50 value of 29.00 μM (95% CI, 23.46–35.86 μM), which is higher than that of the wild-type virus, with an EC 50 value of 15.74 μM (95% CI, 11.82–20.96 μM; Fig. 2d ). Compared with its wild-type counterpart, recombinant H5N1 virus with the PB1-V43I mutation showed reduced sensitivity to increasing concentrations of ribavirin in MDCK cells ( Fig. 2e ). Importantly, the PB1-V43I mutation did not significantly reduce the polymerase activity of the H5N1 polymerase complex (wild-type polymerase activity is 12.64±0.5366 (mean firefly/renilla luciferase ratio±s.d. ), whereas for V43I mutant is 12.98±0.3647; Supplementary Fig. 4a ). PB1 of IAV encodes three polypeptides, PB1, PB1-F2 and the recently identified N40 protein [22] . The PB1-V43I mutation in PB1 protein would lead to an amino-acid change (V3I) in the N40 protein but not in the PB1-F2 protein, as CAG in PB1 and CAA in PB1-F2 both encode glutamine. To ensure that the phenotype we observed was purely derived from the PB1-V43I mutation but not due to the V3I mutation in the N40 protein, we eliminated the expression of N40 protein by introducing a PB1-M40L mutation to remove the start codon of PB1-N40 of the VN04 polymerase complex. This approach allows direct assessing of the effect of the PB1-V43I mutation in the PB1 protein without being confounded by the V3I mutation in the N40 protein. VN04 polymerase complex was selected over the Wuhan95 polymerase complex to study the effect of PB1-N40, as the V43I mutation did not cause significant reduction in VN04 polymerase activity ( Supplementary Fig. 4a ) but would reduce the Wuhan95 polymerase activity by ~50%. 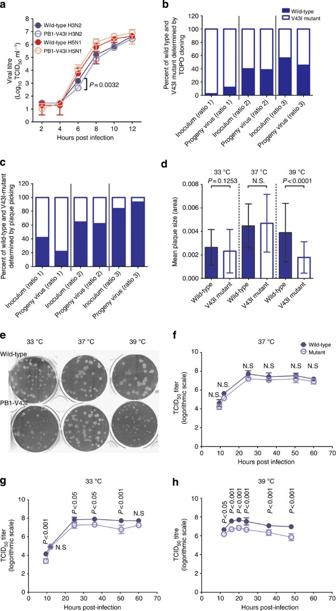Figure 3: Replication kinetics of wild-type and PB1-V43I viruses under competition or suboptimal temperatures. (a) One-step growth kinetics of wild-type and PB1-V43I H3N2 and H5N1 viruses using MOI 1–2 TCID50per cell in MDCK cells. Viral supernatants were collected every 2 h post infection and viral titres (mean±s.d. log10TCID50per ml) from triplicates were shown. The replication kinetics has been repeated three times for the H3N2 wild-type and PB1-V43I viruses and once for the H5N1 wild-type and PB1-V43I viruses. (b) Competitive replication of wild-type and PB1-V43I-mutant virusesin vitro. Wild-type and PB1-V43I viruses were premixed at different ratios before infection of MDCK cells. To determine the actual ratio in both the premixed (inoculum) and the viral supernatant after incubation for 2 days (progeny virus), clonal sequencing was performed to determine the ratio between Wuhan95 wild-type and PB1-V43I viruses. (c) As an alternative, in a separate experiment, instead of clonal sequencing, plaque assay was performed for the inoculums and passage-one viral supernatant after incubation for 2 days. Then, 32 clones were picked for each of the three inoculums and three corresponding passage-one viral cultures for viral RNA isolation and RT–PCR of thePB1gene region that can distinguish wild-type virus from its V43I-mutant counterpart. The actual ratio in the inoculums and the viral supernatant was shown in the same manner. (d) The mean plaque sizes formed by the Wuhan95 wild-type and PB1-V43I viruses incubated at different temperatures. Wild-type or PB1-V43I-mutant viruses were used to infect MDCK monolayers in triplicates and were incubated under 0.5% agar overlay for 48 h at 33, 37 or 39 °C. The experiments were repeated independently twice and one representative result was shown. (e) Picture taken for the one representative plaque assay experiment performed for wild-type and V43I-mutant viruses at the three temperatures. (f) Growth curve of wild-type and V43I-mutant Wuhan95 viruses performed at 37 °C, (g) 33 °C and (h) 39 °C. Forf–h, viral titres (mean±s.d. log10TCID50per ml) from quadruplicated wells were shown. Three independent experiments were performed, with one representative experiment being displayed.Pvalues were based on two-way analysis of variance test with Bonferroni post tests. N.S., not statistically significant. The introduction of the M40L mutation in the absence or presence of the PB1-V43I mutation was observed to reduce the polymerase activity to 80.21 or 64.19%, respectively ( Supplementary Table 3 ). Comparing with the VN04 polymerase complex containing the PB1-M40L mutation, the combination of the M40L and V43I PB1 mutations retains resistance to ribavirin ( Supplementary Fig. 4b ). In summary, we identified a single V43I mutation in PB1 protein that confers resistance to ribavirin in both the human-origin Wuhan95 and the avian-origin VN04 polymerase complexes. The PB1-V43I mutation introduced in recombinant Wuhan95 or VN04 viruses similarly confers to reduced sensitivity to ribavirin. Fitness of the PB1-V43I-recombinant virus in vitro To compare the viral fitness of the PB1-V43I variant with its wild-type counterpart in vitro , we determined the single-cycle replication kinetics of the H3N2- and the H5N1-recombinant wild-type and PB1-V43I viruses in MDCK cells. For the H3N2-recombinant viruses, the PB1-V43I virus replicated to half a log lower titre than that of the wild-type virus at 6 h post infection; however, both viruses reached comparable titres after 8 h post infection ( Fig. 3a ). For the H5N1-recombinant viruses, both the wild-type and the PB1-V43I viruses replicated to comparable titres ( Fig. 3a ). Overall, the results of replication kinetics correlated with the polymerase activity of the H3N2 and H5N1 polymerase complexes as described previously. Figure 3: Replication kinetics of wild-type and PB1-V43I viruses under competition or suboptimal temperatures. ( a ) One-step growth kinetics of wild-type and PB1-V43I H3N2 and H5N1 viruses using MOI 1–2 TCID 50 per cell in MDCK cells. Viral supernatants were collected every 2 h post infection and viral titres (mean±s.d. log 10 TCID 50 per ml) from triplicates were shown. The replication kinetics has been repeated three times for the H3N2 wild-type and PB1-V43I viruses and once for the H5N1 wild-type and PB1-V43I viruses. ( b ) Competitive replication of wild-type and PB1-V43I-mutant viruses in vitro . Wild-type and PB1-V43I viruses were premixed at different ratios before infection of MDCK cells. To determine the actual ratio in both the premixed (inoculum) and the viral supernatant after incubation for 2 days (progeny virus), clonal sequencing was performed to determine the ratio between Wuhan95 wild-type and PB1-V43I viruses. ( c ) As an alternative, in a separate experiment, instead of clonal sequencing, plaque assay was performed for the inoculums and passage-one viral supernatant after incubation for 2 days. Then, 32 clones were picked for each of the three inoculums and three corresponding passage-one viral cultures for viral RNA isolation and RT–PCR of the PB1 gene region that can distinguish wild-type virus from its V43I-mutant counterpart. The actual ratio in the inoculums and the viral supernatant was shown in the same manner. ( d ) The mean plaque sizes formed by the Wuhan95 wild-type and PB1-V43I viruses incubated at different temperatures. Wild-type or PB1-V43I-mutant viruses were used to infect MDCK monolayers in triplicates and were incubated under 0.5% agar overlay for 48 h at 33, 37 or 39 °C. The experiments were repeated independently twice and one representative result was shown. ( e ) Picture taken for the one representative plaque assay experiment performed for wild-type and V43I-mutant viruses at the three temperatures. ( f ) Growth curve of wild-type and V43I-mutant Wuhan95 viruses performed at 37 °C, ( g ) 33 °C and ( h ) 39 °C. For f – h , viral titres (mean±s.d. log 10 TCID 50 per ml) from quadruplicated wells were shown. Three independent experiments were performed, with one representative experiment being displayed. P values were based on two-way analysis of variance test with Bonferroni post tests. N.S., not statistically significant. Full size image The stability of the PB1-V43I mutation in the H3N2 virus after five passages in MDCK cells was confirmed by Sanger sequencing. We observed that the V43I mutation was stably maintained; however, a subpopulation of A370V PB1 mutation was noted at passage 5 by Sanger sequencing and was further confirmed by clonal sequencing (46.2%). No additional mutation was noted in the other seven segments of the PB1-V43I virus after five passages in MDCK cells by Sanger sequencing. The effect of the A370V mutation was assessed using the mini-genome assay. 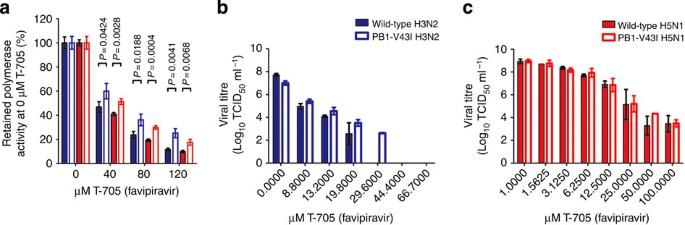Figure 4: Effect of PB1-V43I mutation on favipiravir sensitivities. (a) Sensitivity of the PB1-V43I mutation in Wuhan95 and VN04 polymerase complexes to favipiravir (0–120 μM) was determined using the mini-genome assay. (b) Favipiravir dose–response curve in MDCK cells using the recombinant H3N2 wild-type and the PB1-V43I viruses (MOI=0.1). (c) Favipiravir dose–response curve in MDCK cells using the recombinant H5N1 wild-type and the PB1-V43I viruses (MOI=0.001). The supernatant was harvested at 48 h post infection for titration. The viral titres (mean±s.d. log10TCID50per ml) from triplicates are shown. Student’st-test was performed to calculate thePvalues. As observed previously, the V43I mutation alone reduced polymerase activity by 1.46 fold when compared with that of the wild-type virus; however, the combination of V43I and the A370V mutations increased the polymerase activity by 1.66 fold when compared with that of the wild-type virus ( Supplementary Table 4 ). Therefore, the A370V mutation may play a compensatory role to rescue the decreased polymerase activity caused by the V43I mutation in the Wuhan95 polymerase complex. We further conducted a direct competition assay between the PB1-V43I variant and its wild-type counterpart in vitro ( Fig. 3b ). MDCK cells were infected at MOI 0.1 by a mixture of the H3N2 wild-type and the PB1-V43I variant at three different ratios. The three ratios between the wild-type and V43I-mutant viruses were intended to be at 25:75%, 50:50% and 75:25%; however, the exact ratios were confirmed by clonal sequencing of the inoculum to be at 2.4:97.6%, 40:60% and 56.3:43.8%. The ratios between the wild-type and the PB1-V43I variant in the viral progenies at 48 h post infection, as determined by TOPO cloning of the reverse transcription PCR (RT–PCR) product of viral RNA extracted from the virus supernatant, were comparable to that of the inoculums ( Fig. 3b ), suggesting that the wild-type and the PB1-V43I viruses possess comparable viral fitness in vitro under minimal selection pressure. To further verify the competitive fitness between the Wuhan wild-type and the PB1-V43I-mutant viruses, MDCK cells were infected at MOI=0.1 with mixtures of the two viruses 41.9:58.1%, 64.5:35.5% and 83.9:16.1% (verified by RT–PCR and sequencing of the PB1 gene flanking the V43I region from plaques formed by the inoculums). Culture supernatants were harvested at 48 h post infection. The post-infection ratio between the Wuhan wild-type and PB1-V43I-mutant viruses were determined by RT–PCR and sequencing of the PB1 gene flanking the V43I region with 32 picked plaques per reaction. Similar to the previous observation, the ratio of wild-type and V43I mutant remains comparable before and after one passage in MDCK cells ( Fig. 3c ), suggesting that the PB1-V43I mutation did not compromise viral fitness under direct competition assay with the wild-type virus. To assess whether the wild-type and PB1-V43I viruses exhibited similar viral fitness at suboptimal conditions, we determined the plaque sizes of the wild-type and the PB1-V43I viruses at 33, 37 and 39 °C ( Fig. 3d ). The two viruses formed comparable sizes of plaques at 33 or 37 °C, but the wild-type virus formed significantly larger plaques than that of the PB1-V43I virus at 39 °C ( Fig. 3e ). In addition, we determined the viral replication kinetics with an MOI of 0.01 of the Wuhan wild-type and V43I-mutant viruses at 33, 37 and 39 °C in MDCK cells. Comparable virus replication efficiency was observed for the Wuhan wild-type and PB1-V43I-mutant viruses at 37 °C ( Fig. 3f ), while minor differences in replication efficiency was noted at 33 °C ( Fig. 3g ). The difference in replication efficiency between the wild-type and PB1-V43I viruses was most noticeable at 39 °C, as the V43I-mutant virus replicated to lower viral titres while compared with its wild-type counterpart at all six time points examined ( Fig. 3h ). The result suggests that the wild-type virus may possess a replicative advantage over the PB1-V43I virus under the suboptimal condition of higher temperature. PB1-V43I confers reduced favipiravir sensitivity To further investigate the molecular mechanism for the increased resistance to ribavirin displayed by the PB1-V43I mutation, we applied the polymerase-based mini-genome assay to assess whether the mutation would similarly confer reduced sensitivity to another purine analogue, favipiravir, for which no IAV-resistant variants has been reported. PB1-V43I mutation in the polymerase complex of either Wuhan95 (H3N2) or VN04 (H5N1) exhibited decreased sensitivity to favipiravir compared with that of the wild-type polymerase complexes, although the difference is not as significant as observed for ribavirin ( Fig. 4a ). Applying the mini-genome assay, the calculated EC 50 as determined of the PB1-V43I H3N2 and PB1-V43I H5N1 viruses was shown to be 49.11 μM (95% CI, 41.05–58.76 μM) and 59.66 μM (95% CI, 41.00–86.81 μM), respectively, while those of the H3N2 and H5N1 wild-type polymerases were determined to be only 27.88 μM (95% CI, 22.28–34.88 μM) and 40.08 μM (95% CI, 33.84–47.47 μM), respectively. Figure 4: Effect of PB1-V43I mutation on favipiravir sensitivities. ( a ) Sensitivity of the PB1-V43I mutation in Wuhan95 and VN04 polymerase complexes to favipiravir (0–120 μM) was determined using the mini-genome assay. ( b ) Favipiravir dose–response curve in MDCK cells using the recombinant H3N2 wild-type and the PB1-V43I viruses (MOI=0.1). ( c ) Favipiravir dose–response curve in MDCK cells using the recombinant H5N1 wild-type and the PB1-V43I viruses (MOI=0.001). The supernatant was harvested at 48 h post infection for titration. The viral titres (mean±s.d. log 10 TCID 50 per ml) from triplicates are shown. Student’s t -test was performed to calculate the P values. Full size image We then examined whether the PB1-V43I mutation affects the sensitivity of recombinant H3N2 or H5N1 viruses to favipiravir in MDCK cells. The wild-type H3N2 virus has an EC 50 value of 10.98 μM (95% CI, 6.93–17.41 μM) compared with a 2.24-fold increase in EC 50 to 24.61 μM (95% CI, 17.65–34.32 μM) in the PB1-V43I mutant when infected at a MOI of 0.1 ( Fig. 4b ). Although there is a reduction in favipiravir sensitivity observed for the VN04 PB1-V43I polymerase complex by the mini-genome assay, the recombinant H5N1 VN04 virus carrying the PB1-V43I mutation (EC 50 =17.85; 95% CI, 11.69–27.27 μM) did not show significant resistance to favipiravir while compared with its wild-type counterpart (EC 50 =18.97; 95% CI, 12.26–29.38 μM) at MOI of 0.001 ( Fig. 4c ). Overall, we identified that the V43I mutation confers reduced sensitivity to both ribavirin ( Fig. 2d ) and favipiravir at the polymerase level ( Fig. 4a ). PB1-V43I confers increased guanosine selectivity As ribavirin is a purine analogue, it is possible that the PB1-V43I mutant, which exhibited altered selectivity to ribavirin, would possess altered binding affinity for GTP or ATP. We evaluated the effect of guanosine treatment on the polymerase activity of both wild-type PB1 and PB-V43I proteins in IAV mini-genome assay. The VN04 polymerase complex was used for the assay as the V43I mutation does not significantly decrease its activity. We observed that an increasing concentration of guanosine leads to reduced polymerase activity (as reflected by the expressed firefly luciferase activity) for both the wild-type as well as PB1-V43I polymerase complexes ( Fig. 5a ). The reduction in polymerase activity is likely through the biased intracellular nucleoside triphosphate (NTP) concentrations, as the addition of 25–500 μM guanosine to the Jurkat cells has been reported to increase intracellular GTP but deplete ATP concentrations [23] . Interestingly, we observed that the PB1-V43I protein exhibited more significant reduction in polymerase activity under increasing concentration of guanosine ( Fig. 5a ), suggesting that the PB1-V43I showed increased selectivity for nucleosides over the wild-type PB1 protein under the biased intracellular NTP concentrations. The observed greater reduction in the polymerase activity (as reflected by expressed firefly luciferase activity) by the PB1-V43I protein under high guanosine concentrations (leading to biased intracellular NTP concentration) can be due to direct inhibition of RdRP as a result of increased nucleoside selectivity, or due to mutagenesis effect under the biased intracellular NTP concentration, leading to increased deleterious mutations in the luciferase mRNA and the synthesis of non-functional luciferase proteins. To clarify the potential mechanism, we quantified the firefly luciferase mRNA copy numbers from cells co-transfected with the PB1 plasmid carrying the V43I mutation under high guanosine concentrations. The reduced polymerase activity (as reflected by reduced firefly luciferase activity) was correlated with lower firefly luciferase mRNA levels from cells co-transfected with the PB1 plasmid carrying the V43I mutation ( Fig. 5b ). This observation further supports that the reduced polymerase activity is through decreased RNA synthesis. However, we cannot rule out the possibility that the reduced luciferase mRNA copy numbers can also be explained by reduced promoter binding, cap binding or cap cleavage by the viral polymerase. 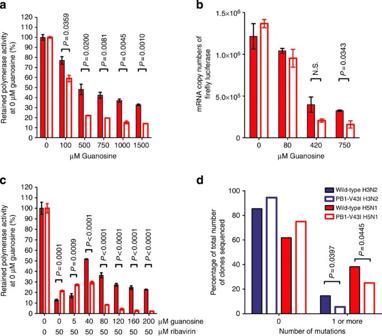Figure 5: Effects of PB1-V43I mutation on guanosine selectivity and mutational frequencies. (a) Effect of increasing concentrations of guanosine on VN04 wild-type or PB1-V43I polymerase complex using mini-genome assay.Pvalues are based on Student’st-test. The error bars denote s.d. calculated for samples performed in triplicates. The experiment was repeated twice independently. (b) Firefly luciferase mRNA expression (copy numbers) under increasing concentration of guanosine.Pvalues are based on Student’st-test. (c) Guanosine and ribavirin competition assay to determine the effect of guanosine in reversing the inhibitory effects of ribavirin on wild-type versus PB1-V43I polymerases.Pvalues are based on Student’st-test. The mean±s.d. relative polymerase activities under different concentrations of ribavirin and guanosine were determined from triplicate samples. The experiment was repeated twice independently. (d) Mutation frequencies of recombinant Wuhan95 or VN04 wild-type and PB1-V43I viruses in theHAgene were determined by clonal sequencing. Data were expressed as the percentage of clones with 0 or ≥1 mutations in theHAgene. One of the three independently repeated experiments is shown. Fisher’s exact test was performed to determine thePvalues. Figure 5: Effects of PB1-V43I mutation on guanosine selectivity and mutational frequencies. ( a ) Effect of increasing concentrations of guanosine on VN04 wild-type or PB1-V43I polymerase complex using mini-genome assay. P values are based on Student’s t -test. The error bars denote s.d. calculated for samples performed in triplicates. The experiment was repeated twice independently. ( b ) Firefly luciferase mRNA expression (copy numbers) under increasing concentration of guanosine. P values are based on Student’s t -test. ( c ) Guanosine and ribavirin competition assay to determine the effect of guanosine in reversing the inhibitory effects of ribavirin on wild-type versus PB1-V43I polymerases. P values are based on Student’s t -test. The mean±s.d. relative polymerase activities under different concentrations of ribavirin and guanosine were determined from triplicate samples. The experiment was repeated twice independently. ( d ) Mutation frequencies of recombinant Wuhan95 or VN04 wild-type and PB1-V43I viruses in the HA gene were determined by clonal sequencing. Data were expressed as the percentage of clones with 0 or ≥1 mutations in the HA gene. One of the three independently repeated experiments is shown. Fisher’s exact test was performed to determine the P values. Full size image We then evaluated the effect of guanosine for both the wild-type PB1 and PB1-V43I proteins in the presence of ribavirin. We showed that guanosine (20 μM) can restore Wuhan95 replication in the presence of ribavirin (40 μM; Fig. 1b ). As we observed previously, the wild-type PB1 activity inhibited by ribavirin (120 μM) can be partially rescued at low concentrations of guanosine (≤40 μM); however, the PB1 activity was significantly reduced under higher guanosine concentrations, likely through the biased NTP concentrations ( Fig. 5c ). In contrast, increased guanosine (≤40 μM) did not reverse the inhibitory effects of ribavirin on PB1-V43I as efficiently as that on the wild-type PB1 protein, suggesting that the PB1-V43I protein may possess a reduced affinity to GTP at low concentrations of guanosine. Under higher guanosine concentrations, at which a biased intracellular NTP concentration is likely present, the PB1-V43I protein exhibited further reduced polymerase activity than that of the wild-type PB1 protein. Overall, the results suggest that the V43I mutation increased the nucleoside selectivity of the PB1 protein. PB1-V43I reduces H3N2 and H5N1 mutational frequencies Resistant variants selected by ribavirin of the Piconaviridae and Togaviridae families have been reported to possess altered polymerase fidelity [9] , [11] , [20] . To confirm that the PB1-V43I mutation conferring ribavirin resistance would also affect IAV polymerase fidelity, clonal sequencing was performed to calculate the mutational frequency between the wild-type and the PB1-V43I viruses. The HA gene of the recombinant Wuhan95 (H3N2) or VN04 (H5N1) wild-type and PB1-V43I viruses that were passaged twice in MDCK cells was analysed. The mutation frequency of the H3N2 wild-type virus was calculated to be higher compared with that of the PB1-V43I virus by a factor ranging from 0.98 to 3.12 in three independent experiments ( Fig. 5d ; Supplementary Table 5 ). 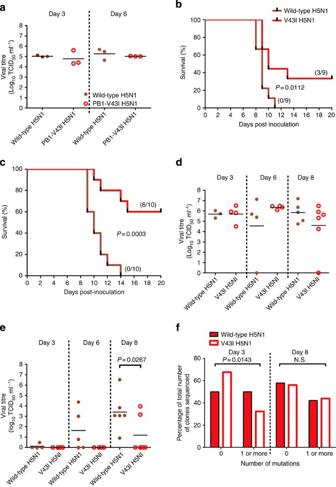Figure 6:In vivocharacterization of wild-type and PB1-V43I-mutant H5N1 viruses. (a) Viral titres of lung homogenate of mice inoculated with 100 p.f.u. of wild-type and PB1-V43I H5N1 viruses at 3 and 6 days post inoculation. (b) Survival curves of mice (N=9 per group) inoculated with 100 p.f.u. of H5N1 wild-type or PB1-V43I viruses. Log-rank (Mantel–Cox) test confirmed the statistically significant differences in mouse survival after infection with the H5N1 wild-type and PB1-V43I viruses. (c) Survival curves of mice (N=10 per group) inoculated with 10 p.f.u. of H5N1 wild-type or PB1-V43I viruses. Viral titres (log10TCID50per ml) in mouse lungs (d) and brain (e) homogenate after being inoculated with 10 p.f.u. of H5N1 wild-type and PB1-V43I viruses at 3, 6 and 8 days post inoculation were determined. (f) Mutation frequencies in theHA1gene (nucleotides 57–978) of H5N1 wild-type and PB1-V43I viruses from mouse lungs collected at days 3 and 8 post inoculation. Results were expressed as the percentage of clones with 0 or ≥1 mutations in theHA1gene. Fisher’s exact test was performed to determine thePvalue. A similar trend was observed when we calculated the mutational frequency in the NA gene of the H3N2 wild-type and the PB1-V43I viruses; the wild-type H3N2 virus (7.06 mutations per 10 4 nucleotides) showed 1.49-fold higher mutational frequency than that of the PB1-V43I virus (4.75 mutations per 10 4 nucleotides) ( Supplementary Table 6 ). Since ribavirin may act as a mutagen for IAV RdRP, a reduced mutation frequency would be expected for the PB1-V43I virus after passaging in the presence of ribavirin. Therefore, we determined the mutational frequencies of the wild-type and the PB1-V43I viruses after one passage in the presence of 66.6 μM ribavirin in MDCK cells. After 48 h, viral supernatant was collected to determine the mutational frequencies in the HA gene by clonal sequencing ( Supplementary Table 7 ). We observed that in the presence of ribavirin, the wild-type virus (5.53 mutations per 10 4 nucleotides) exhibited a 1.36-fold higher mutational frequency than that of the PB1-V43I virus (4.08 mutations per 10 4 nucleotides). In addition to applying clonal sequencing, we also directly sequenced the HA gene of plaques formed by the Wuhan wild-type and PB1-V43I viruses in MDCK cells by Sanger sequencing. The wild-type virus (1.67 mutations per 10 4 nucleotides) has 4.76-fold higher mutational frequencies when compared with that of the PB1-V43I mutant (0.35 mutations per 10 4 nucleotides) ( Supplementary Table 8 ). Applying clonal sequencing, the mutational frequency in the HA gene of the recombinant H5N1 virus carrying the PB1-V43I mutation was lower compared with that of its wild-type counterpart by a factor of 1.39–1.55 ( Fig. 5d ; Supplementary Table 9 ). PB1-V43I H5N1 IAV exhibited reduced pathogenicity in mice We evaluated the effect of mutation frequency on viral fitness in vivo using the recombinant H5N1 viruses with or without the PB1-V43I mutation at a challenge dose of 100 p.f.u. ( Fig. 6a,b ) or 10 p.f.u. ( Fig. 6c–e ), respectively. At either challenge dose, both the wild-type and the high-fidelity H5N1 viruses replicated to comparable titres in the mouse lungs on days 3, 6 and 8 (10 p.f.u. only) post inoculation ( Fig. 6a,d ). The PB1-V43I variant was tenfold less lethal than wild-type virus with the MLD 50 (mouse lethal dose) at 31.6 or 3.4 p.f.u., respectively. At an inoculation dose of 100 p.f.u., all mice in the wild-type group had died by day 11 post inoculation compared with five out of nine mice in the PB1-V43I virus group; three out of nine mice with PB1-V43I survived at the end point of the experiment (20 days post inoculation). The difference in lethality between wild-type and PB1-V43I is more pronounced when a lower inoculation dose of 10 p.f.u. was used ( Fig. 6c ). All mice (10 out of 10) in the wild-type group died within 14 days post inoculation, while only 4 of 10 mice died in the PB1-V43I virus group at 20 days post inoculation. To further examine the mechanism of the observed difference in lethality between the wild-type and PB1-V43I mutant, the viral titres in the brain were determined to assess the neurotropism of the wild-type and PB1-V43I viruses ( Fig. 6e ). At day 3 post inoculation with 10 p.f.u. per mouse, there was no detectable virus in the brain. At days 6 and 8, the viral titre in the brain was observed to be higher for the wild-type group compared with the PB1-V43I-mutant group ( t -test, P =0.0267). Figure 6: In vivo characterization of wild-type and PB1-V43I-mutant H5N1 viruses. ( a ) Viral titres of lung homogenate of mice inoculated with 100 p.f.u. of wild-type and PB1-V43I H5N1 viruses at 3 and 6 days post inoculation. ( b ) Survival curves of mice ( N =9 per group) inoculated with 100 p.f.u. of H5N1 wild-type or PB1-V43I viruses. Log-rank (Mantel–Cox) test confirmed the statistically significant differences in mouse survival after infection with the H5N1 wild-type and PB1-V43I viruses. ( c ) Survival curves of mice ( N =10 per group) inoculated with 10 p.f.u. of H5N1 wild-type or PB1-V43I viruses. Viral titres (log 10 TCID 50 per ml) in mouse lungs ( d ) and brain ( e ) homogenate after being inoculated with 10 p.f.u. of H5N1 wild-type and PB1-V43I viruses at 3, 6 and 8 days post inoculation were determined. ( f ) Mutation frequencies in the HA1 gene (nucleotides 57–978) of H5N1 wild-type and PB1-V43I viruses from mouse lungs collected at days 3 and 8 post inoculation. Results were expressed as the percentage of clones with 0 or ≥1 mutations in the HA1 gene. Fisher’s exact test was performed to determine the P value. Full size image The mutational frequencies and genetic diversity of wild-type and PB1-V43I viruses in the mouse lungs were assessed by clonal sequencing at day 3 and day 8 post inoculation. At day 3, the mutational frequencies in the HA gene of the wild-type H5N1 virus (8.2 mutations per 10 4 nucleotides) was higher than that of the PB1-V43I-mutant virus (4.4 mutations per 10 4 nucleotides) by a factor of 1.86 (Fisher’s exact test, P =0.0143; Fig. 6f ; Table 2 ). However, such a difference was not observed later at day 8 post inoculation (6.6 mutations versus 6.4 mutations per 10 4 nucleotides; Table 2 ). To assess the stability of PB1-V43I in viruses in vivo , sequences of the PB1 segment of viruses collected at day 8 post inoculation were examined by Sanger sequencing and no reversion to wild type was observed, with no additional mutation found in PB1. The comparable mutational frequency between the wild-type and PB1-V43I-mutant viruses in the mouse lungs at day 8 post inoculation could be a result of strong selection pressure posed by host immune response. Overall, our results showed that a single V43I mutation in PB1 protein confers reduced genetic diversity of the H5N1 VN04 virus at an early time point (day 3) but not at later time point (day 8) post inoculation in vivo . This reduced genetic diversity in the mouse lungs at early time point post inoculation was associated with a reduced pathogenicity in mice. Table 2 Mutational frequency of the VN04 wild-type and the PB1-V43I-mutant viruses from mouse lung homogenate collected at 3 and 8 days post inoculation. Full size table The error-prone RdRP assures adaptation and survival of RNA viruses under different selection pressures. Using an IAV RdRP fidelity variant selected with ribavirin, we provide direct experimental evidence that supports the biological significance of viral genetic diversity on IAV pathogenesis. We demonstrate that a single V43I mutation in PB1 protein confers resistance to ribavirin and increased selectivity to nucleoside, leading to a RdRP with increased fidelity and a reduction in population genetic diversity of both seasonal H3N2 (Wuhan95) and highly pathogenic H5N1 (VN04) viruses. The increased RdRP fidelity similarly reduced VN04 virus population genetic diversity in the mouse lungs at day 3 post inoculation without affecting lung virus titres. Such a reduction in virus population genetic diversity attenuated viral lethality by tenfold with decreased viral neurovirulence. We consider that such a difference in diversity might have affected viral pathogenicity at several levels. First, a more diverse viral population would increase the survival possibility by having subpopulations that may escape neutralizing antibodies or specific T-cell response, adapt better to the host replication machinery or expand tissue tropism. The lung titres between mice inoculated with the VN1203 wild-type or the PB1-V43I-mutant viruses were comparable suggesting that the difference in lethality was not due to differences in the replication capability between these two viruses. It was noted that the PB1-V43I VN04 virus showed reduced neurotropism while compared with the VN1203 wild-type virus. Such a difference was previously demonstrated by Pfeiffer et al. [19] and Vignizzi et al. [20] that different virus population may act synergistically and contribute neurovirulence of poliovirus. Furthermore, with the Wuhan wild-type and PB1-V43I viruses, we demonstrated that they differed in the ability in generating monoclonal antibody escape mutants ( Supplementary Fig. 5 ). Further studies would be needed to elucidate the precise mechanism leading to differences in lethality observed with the VN1203 wild-type and PB1-V43I mutants. However, these results provide experimental evidence supporting the role of viral genetic diversity in viral pathogenicity. The reported IAV fidelity variant can be further applied to study viral population dynamics under different selection pressures within and between hosts. The ability to manipulate the RdRP mutational rate has so far been restricted to the non-segmented, positive-sense, single-stranded RNA viruses of the Piconaviridae and Togaviridae families, both with similar polymerase structures. Studies on the high-fidelity variants of poliovirus showed reduced viral pathogenicity in vivo as a result of reduced ability to adapt to the in vivo environment, including the inability to acquire a reversion mutation (back from the introduced attenuating mutation) at permissive temperature [19] or reduced neutrotropism in mice [20] . High-fidelity chikungunya virus, an arbovirus that requires transmission between an invertebrate (mosquito) and a vertebrate host, was shown to replicate to lower viral titres than that of the wild-type virus in both hosts [9] . Interestingly, the viral fitness (replication efficiency) of the wild-type and the high-fidelity viruses in vitro was often comparable or only moderately affected [9] , [19] , [20] . One the other hand, RdRP with increased mutational frequency (low-fidelity RdRP) would also lead to reduced pathogenicity in vivo , as the Coxsackievirus B3 fidelity variant with increased mutation frequency was observed to be attenuated in vivo [24] . Overall, our data and that from others in different virus models support the idea that the RNA viruses replicate within a finely tuned and narrow error threshold to achieve optimal survival, especially under in vivo conditions. Attenuation of virus virulence in vivo without significantly affecting viral replication in vitro would be a desirable property to be included in the future development of live-attenuated vaccines [25] . Structural insights are available for multiple domains derived from the PB2 and PA proteins, but there is limited structural insight available for the PB1 protein that possess the catalytic function for RdRP [26] . So far, it has been demonstrated that the nucleoside analogue favipiravir can induce mutagenesis in the genome of IAV [14] . However, resistance to favipiravir as a mutagen had not been reported hitherto, raising doubts on whether it is technically feasible to obtain a resistant variant to mutagen for IAV RdRP, which has a heterotrimer structure. Through serial passaging of the Wuhan95 virus in the presence of ribavirin, a total of 11 mutations were identified in the PB2, PB1, PA and NP proteins. We have selected the PB1-V43I mutation for further characterization because of its most significantly decreased sensitivity to ribavirin in the mini-genome system. However, we cannot exclude the possibility that some other mutations, alone or in combination, may also alter IAV RdRP fidelity. This was shown to be the case with enterovirus, where both the G64S and A372V mutations were reported to confer the high-fidelity phenotype [10] . The V43I mutation lies within the putative viral RNA-binding domain in the N terminus of PB1 and is generally quite conserved. A blast search among available influenza PB1 sequences at the NCBI Influenza Virus Source identified a total of five isolates possessing the PB1-V43I mutation. Three out of the five identified sequences are avian origins (two highly pathogenic H5N1 from chicken and Muscovy duck and one H3 influenza virus from ruddy turnstone), and the other two are swine (H1N1) origin. The role of this mutation remains to be determined in the adaptation of IAV to different animal species. The mechanism of ribavirin inhibition of IAV replication has not been previously studied in detail, and the only proposed mechanism has been in the direct inhibition of viral RNA synthesis [27] . Here we provide evidence for a novel mechanism that ribavirin is mutagenic in the viral genome, by inducing G-to-A mutation. In addition to ribavirin, we have evaluated the sensitivity of the PB1-V43I mutation with a panel of nucleoside analogues using the mini-genome assay: tubercidin (adenosine analogue), 6-azauridine (uridine), 8-hydroxy-2′-deoxyguanosine (guanosine), acycloguanosine (guanosine), 5-fluorouracil (uridine), favipiravir (guanosine and adenosine) and N4-aminocytidine (cytidine); the V43I mutation only exhibited reduced sensitivity to ribavirin and favipiravir ( Supplementary Figs 6 and 7 ). Because ribavirin and favipiravir are both purine analogues, we then assessed the effect of guanosine on wild-type PB1 and PB1-V43I proteins to investigate the potential molecular mechanisms of V43I mutation on RdRP fidelity. We confirmed the previous observation that the inhibitory effect of ribavirin can be rescued by low concentration of guanosine (≤40 μM). Guanosine treatment at 500 μM in Jurkat cells was reported to increase GTP to 600% and reduced ATP to 40% than that of untreated control cells [23] . While we did not directly measure the intracellular NTP concentration under increasing guanosine treatment, we observed that the PB1-V43I protein is more sensitive than that of the wild-type PB1 protein under high concentrations of guanosine (>40 μM), leading to a reduced firefly luciferase mRNA synthesis, suggesting that the V43I mutation would increase RdRP selectivity for nucleoside under biased NTP concentrations. Applying expressed polymerase proteins in enzyme-based assays to determine the binding affinity of the PB1 protein with V43I mutation to ribavirin and NTP will further clarify the molecular mechanism of fidelity. Overall, a single PB1-V43I mutation was identified to confer resistance to ribavirin and altered selectivity to guanosine for the polymerase complex derived from both human seasonal H3N2 and the avian-origin H5N1 highly pathogenic influenza viruses. Our results suggest that the PB1-V43I mutation reduced PB1-binding affinity for ribavirin and confer to increased selectivity for NTP, which likely serves as the mechanism for the altered RdRP fidelity and reduced mutational frequency. Applying a fidelity variant with reduced mutational frequency, we provide the first experimental evidence for the role of viral genetic diversity in IAV pathogenesis. This model can be applied to the repertoire of well-developed IAV models to further investigate the role of genetic diversity and population dynamics on influenza pathogenesis and transmission. Compounds Ribavirin (Sigma-Aldrich) was dissolved in water to prepare 2 mM stock. Guanosine (Sigma-Aldrich) was first dissolved in dimethylsulphoxide (DMSO) and then diluted with water to 5 mM. Favipiravir (Carbosynth) was dissolved first with DMSO and then diluted in phosphate buffered saline (PBS) to prepare 2 mM stocks. All stocks were aliquoted and stored at −80 °C until used. Viruses and cells MDCK and human embryonic kidney 293T cells were obtained from ATCC and were maintained as described [28] . Recombinant A/Wuhan/359/95 (H3N2) (Wuhan95) and A/Vietnam/1203/04 (H5N1) (VN04) viruses were generated by co-transfecting human embryonic kidney 293T cells (TransIT-LT1; Mirus Bio) with eight plasmids (1 μg each) encoding the eight segmented genome of IAV within the dual promoter pHW2000 vector [28] , [29] , [30] . Recombinant viruses were passaged twice in MDCK cells at MOI=0.001 before used for in vitro and in vivo experiments. Single or multiple point mutants were introduced into the PB1, PB2, PA and NP plasmids using QuikChange Lightning Site-Directed Mutagenesis Kit (Agilent Technologies) or QuikChange Lightning Multi Site-Directed Mutagenesis Kit, respectively. The full genome sequences (eight gene segments) of the recombinant viruses were verified. All work with highly pathogenic H5N1 viruses were conducted in the Biosafety Level-3 laboratory at the LKS Faculty of Medicine, The University of Hong Kong, following approved guidelines. Introducing the PB1-V43I mutation into the VN04 virus was anticipated to reduce viral virulence, as was indeed observed, with viruses with a high-fidelity RdRP exhibiting reduced pathogenicity in the mouse model [9] , [19] , [20] . This experiment therefore is neither a gain-of-function experiment nor one with potential for Dual Use Research of Concern (DURC). Ribavirin and guanosine MTT assays Cell suspensions (200 μl) in culture media are seeded and incubated at 37 °C and 5% CO 2 at a cell density to reach 100% confluence of monolayer of MDCK cells the next day. Dilutions of drugs were performed in twofold serial dilutions with 1.5 mM of ribavirin and 4 mM guanosine with infectious media. Then, culture media were aspirated and washed with PBS once before 200 μl of drug-media mixture was used to incubate the cells for 48 h at 37 °C and 5% CO 2 . Then, MTT was dissolved in DMSO at 1 mg ml −1 . Then, 50 μl of MTT was mixed with 200 μl of OPTI-MEM with minimal phenol red added into the wells. Cells were incubated for 4 h at 37 °C with 5% CO 2 . After 4 h, the MTT mixture was aspirated and replaced with 200 μl of DMSO and 25 μl Sorenson’s buffer at pH 10.5 that consists of 0.1 M glycine and 0.1 M NaCl. The plate was then incubated at room temperature for 5 min. The optical density of each well was detected by a plate reader at 630 nm of reference wavelength and 570 nm of test wavelength. As an alternative method to measure cytotoxicity, CellTiter-Glo Luminescent Cell Viability Assay (Promega) was used according to manufacturer’s instructions after the removal of cell media. The luminescent signal is proportional to the amount of ATP present, which is directly proportional to the number of cells present in culture. Serial passaging of the Wuhan95 virus with ribavirin The concentration of ribavirin that reduced Wuhan95 viral titre as determined by TCID 50 and real-time PCR of M gene by ~75% (logarithmic scale) was pre-determined to be 35–40 μM ( Supplementary Fig. 1a,b ). For every passage, MDCK cells were infected with Wuhan95 at an MOI of 0.01 TCID 50 per cell in six replicates. After incubation, cells were washed with PBS, and overlaid with infection medium (with 1 μg ml −1 TPCK-trypsin) containing 35 μM ribavirin for passages 1–11 and 40 μM for passages 12–17 for 3 days, at which point viral supernatant with cellular debris removed by centrifugation was collected and stored at −80 °C for virus titration. The TCID 50 viral titres were determined as described above. Passage of four of the six replicates was stopped when no virus could be detected by the TCID 50 assay (detection limit: 10 1.789 TCID 50 per ml). Plaque assay Confluent MDCK cells seeded in six-well plates were washed with PBS twice. Serial tenfold dilutions of virus were performed with infection media, and washed cells were inoculated with 1 ml of the diluted virus. After 1 h incubation at 37 °C, inoculums were removed, washed with PBS and overlaid with infection medium containing 1% agarose and 1 μg ml −1 TPCK-trypsin. Plaques were visualized after incubation at 37 °C for 3 days by overnight fixation with 4% formaldehyde in PBS followed by staining with 0.2% crystal violet. To compare the differences between wild-type and PB1-V43I mutant to replicate at suboptimal temperatures (33 and 37 °C), 0.5% agarose was used and triplicates of six wells were used to incubate for 48 h at these temperatures. After formaldehyde fixation, the plates were scanned using Scanjet 5590, and the mean plaque size was determined by measuring the areas of more than 100 plaques from the triplicates of wells. Student’s t -test was used for statistical differences between groups. TCID 50 determination Confluent MDCK cells were seeded in 96-well plates. Cells were washed twice with PBS and overlaid with 100 μl of infection media supplemented with 1 μg ml −1 TPCK-treated trypsin (for H3N2 virus only). Serial half-log dilutions, from 10 −0.5 to 10 −8 , were performed in 96-well plates, and 35 μl of the virus dilutions was added onto the MDCK-seeded plates in quadruplicate. After 3 days, a hemagglutination assay was performed using 0.5% turkey red blood cells in PBS to determine TCID 50 as reported by Reed and Muench [31] . The detection limit is 10 1.789 TCID 50 per ml. Cell-based plaque reduction assays Cell-based plaque reduction assay was used to select variants from the whole viral population displaying resistance to ribavirin. Confluent MDCK cells seeded in six-well plates were infected with 200 p.f.u. of virus per well and incubated for 1 h at 37 °C and 5% CO 2 . After incubations, cells were washed with PBS and replenished with infection medium containing 1% agarose, TPCK-trypsin and increasing concentrations of ribavirin. Two days post infection, infectious media containing neutral red and agarose were used to stain infected cells for plaque picking on the third day. MTT assay Confluent MDCK cells seeded in 96-well plates were overlayed with 200 μl compounds serial twofold diluted with infection media (ribavirin (dose range, 10 μM–1 mM) and guanosine (dose range, 10 μM–10 mM)). MTT was dissolved in DMSO at 1 mg ml −1 , and 50 μl of MTT was mixed with 200 μl of OPTI-MEM for a final concentration of 200 μg ml −1 MTT. After 48 h incubation at 37 °C and 5% CO 2 , the drug-media mixture was aspirated and replaced with 250 μl of MTT in OPTI-MEM. Cells were incubated for 4 h at 37 °C with 5% CO 2 . After 4 h, the MTT mixture was aspirated and replaced with 200 μl of DMSO and 25 μl Sorenson’s buffer at pH 10.5 that consists of 0.1 M glycine and 0.1 M NaCl. The plate was then incubated at room temperature for 5 min. The optical density (absorbance) of each well was detected by a plate reader at 630 nm of reference wavelength and 570 nm of test wavelength. One-step growth kinetics One-step growth curves were determined for wild-type and the PB1-V43I-mutant viruses in MDCK cells. Confluent cell monolayer seeded in 24-well plates was infected with viruses at a MOI of ~2 TCID 50 per cell. After incubation, the cells were washed once with 0.85% aqueous NaCl solution at pH 2.4–2.5 followed by one wash with PBS. Supernatants were collected 2, 4, 6, 8, 10 and 12 h post infection. TCID 50 viral titration was then performed. Direct competition assay Wild-type and PB1-V43I-mutant viruses were mixed into three different ratios to infect MDCK cells in triplicate wells in 6-well plates at an MOI of 0.1. Total RNA was extracted from the inoculum (0 h post infection) and viruses were collected from MDCK cells at 48 h post infection using RNEasy kit (Qiagen). A 382-bp PCR product was amplified (One-step RT-PCR; Qiagen) using specific primers (forward, 5′-AAAGCAGGCAAACCATTTGA-3′ and reverse, 5′-TGTCCACCCTTGTTTGTTGA-3′). The RT–PCR product was cloned into the pCR4-TOPO vector (Invitrogen). Plasmid DNA was isolated (Miniprep; Qiagen), and a total of 57–140 clones were sequenced using the T3 primer, covering the nucleotide encoding amino-acid residue 43. As an alternative method of measuring the actual ratio in the inoculums and passage-one viral progeny cultures, plaque assays were performed for the isolation of 32 clones for each population, and then RT–PCR of the PB1 gene region containing the V43I signature mutation was performed separately using the above primers to distinguish the wild type from the mutant viruses using Sanger sequencing. Real-time PCR of mRNA extracted from mini-genome assays Two out of three replicates of transfected 293T cells were lysed with RLT buffer, and total RNA was extracted with RNeasy kit (Qiagen). To remove potential DNA contamination from plasmids used to transfect the cells, 5 μg of extracted RNA was incubated for 3 h at 37 °C with a mixture of 2 U Turbo DNA-free DNase (Applied Biosystems) and 2 U DpnI (New England Biolabs). Reverse transcription using High-fidelity Transcriptor Kit (Roche) was then performed with standardized amount of RNA using Oligo(dT) 18 . Synthesized complementary DNA was diluted five times. Real-time PCR of firefly and renilla luciferase genes were performed on a Roche 480 Lightcycler instrument using the SYBR Green I Master Mix (Roche), following the manufacturer’s instructions. In each reaction, 5 μl of cDNA, 10 μl of the probe master mix (2 × ), 0.5 μM each of forward and reverse primers and water was used. Plasmid DNA containing the firefly and renilla luciferase genes was used as standard diluted serially at tenfold. The reaction has a hot start step at 95 °C for 10 min for 1 cycle, 45 cycles of denaturation at 95 °C for 10 s, annealing at 62 °C for 10 s and extension at 72 °C for 40 s. Sensitivity of RdRP to nucleoside analogues Sub-confluent monolayer of 293T cells seeded in 24-well plates was pretreated with 25, 50 and 75 μM of ribavirin, 40, 80 and 120 μM favipiravir (Carbosynth) or 80, 420 and 750 μM guanosine (Sigma-Aldrich) for 2 h before transfection. Other nucleoside analogues (5-azauridine, acyclocytidine, 5-fluorouracil, N4-aminocytidine, turbicidine and 8-hydroxy-2′-deoxyguanosine) were used at the indicated concentrations. Cells were then co-transfected (Mirus Bio) with pHW2000 plasmids encoding the PB2 , PB1 , PA and NP genes (250 ng each for 24-well plates, respectively) plus reporter plasmid (firefly luciferase flanked by the noncoding region of M gene segment of IAV driven by human polymerase I promoter; 125 ng for 24-well plates, respectively) [31] and renilla luciferase reporter plasmid driven by CMV promoter for transfection control (2.5 ng for 24-well plates, respectively). After 24 h incubation at 37 °C with 5% CO 2 , cell extracts were prepared in 250 μl lysis buffer and luciferase levels were measured using a Glomax microplate luminometer (Promega). Experiments were independently repeated three times. Ribavirin and favipiravir dose–response assays in MDCK cells Confluent monolayer of MDCK cells seeded in 24-well plates was washed twice with PBS or infectious media and then pretreated with specified concentrations of ribavirin or favipiravir diluted with infection media for 5 h at 37 °C with 5% CO 2 . Cells were then infected with recombinant Wuhan95 or VN04 wild-type or PB1-V43I-mutant viruses at an MOI of 0.1 for both drugs (Wuhan95), 0.1 for ribavirin (VN04) and 0.001 for favipiravir (VN04) and incubated for 1 h. After 1 h, infected cells were washed with PBS and overlaid with infection media of specified concentrations of ribavirin or favipiravir, and further incubated for 48 h. Then, viral supernatant was collected and titrated by the TCID 50 method as described above. No cytotoxicity in MDCK cells was observed by Baranovich et al. [14] at a concentration as high as 1 mM. To quantify the luciferase mRNA copy numbers by quantitative real-time PCR, 293T cells transfected with wild-type or PB1-V43I polymerase complexes under increasing concentration of guanosine were lysed to extract total RNA using RNEasy kit (Qiagen). Reverse transcription was performed with High-fidelity Transcriptor Kit (Roche) using oligo(dT) 18 . Real-time PCR was performed with LighCycler 480 according to manufacturer’s instructions, using primers for firefly luciferase 5′-CATCTTTGGCAACCAGATCA-3′ and 5′-ATGGTCTTTCCATGCTCCAG-3′. Mutational frequency determination by TOPO cloning RNA (20–130 ng) extracted using RNeasy Mini Kit (Qiagen) was used for reverse transcription using Transcriptor High Fidelity cDNA Synthesis Kit (Roche), using random hexamer for cDNA synthesis. Amplification of HA gene was performed by using 10 μl of cDNA in 100 μl reaction using Expand High Fidelity PCR System (Roche) with forward and reverse primers: Wuhan95 (H3N2): 5′-GGTTTTCGCTCAAAAACTTCC-3′ and 5′-GTTTCCCGTTGATTTGGTTG-3′; VN04 (H5N1) 5′-ACCATGCAAACAACTCGACA-3′ and 5′-GCTATTTCTGAGCCCAGTCG-3′. Gel-purified PCR product (24–33 ng) was cloned into pCR4-TOPO vector using TOPO TA Cloning Kit (Life Technologies). Triplicates of 32–48 clones for each of wild-type or PB1-V43I virus were picked and grown in Luria Broth with ampicillin. Clones were sequenced using ABI Prism 3700 sequence analyzers (Applied Biosystems). Pathogenicity of VN04 wild-type and V43I viruses in mice The animal experiments were conducted at the Biosafety Level-3 facility at the LKS Faculty of Medicine, The University of Hong Kong, under applicable guidelines and ethics approved by the Committee on the Use of Live Animals in Teaching and Research (CULATR). To determine the MLD 50 of VN04 wild-type and PB1-V43I viruses, 6-week-old female BALB/c mice were anaesthetized with ketamine and xylazine and inoculated intra-nasally with tenfold serial-diluted wild-type or the PB1-V43I viruses in 25 μl of PBS. To determine the survival curve, groups of mice were inoculated with wild-type or PB1-V43I viruses at 100 or 10 p.f.u. per mice in 25 μl of PBS. Additional mice were inoculated with 100 or 10 p.f.u. of viruses and were killed at day 3, 6 or 8 to collect mouse lungs and brains to determine viral replication and tissue tropism in vivo . Clinical signs were monitored daily. Mice that developed neurological signs such as paralysis or lost over 25% of their original weight were killed. Death and disease signs, as well as weight loss, were recorded daily for 20 days. Log-rank test was performed to compare the survival rate of mice inoculated with the VN04 wild-type and PB1-V43I-mutant viruses. Calculation of mutational frequency and statistical test Sequences were assembled using SeqMan software (DNASTAR Lasergene) with sequence reads in opposite overlapping directions. Alignment was made and mutational frequency was determined using BioEdit and the SeqMan software (DNASTAR Lasergene). Mutational frequency was determined by dividing the number of sites of single nucleotide polymorphism by the total number of nucleotides sequenced. To determine whether the difference among wild-type and PB1-V43I viruses is statistically significant for at least one of the experiments, a 2 × 2 contingency table was formulated comparing the categories of the number of sequences with no mutation and those with at least one mutation. Fisher’s exact test was used to compute the P value from the contingency table. To determine the EC 50 or CC 50 values, the dose–response curves were fitted by non-linear regression, with the variable slope model using GraphPad Prism and the 95% confidence intervals calculated accordingly. How to cite this article: Cheung, P. P. H. et al. Generation and characterization of influenza A viruses with altered polymerase fidelity. Nat. Commun. 5:4795 doi: 10.1038/ncomms5795 (2014).